Self-sustained oscillations of a torsional SQUID resonator induced by Lorentz-force back-action For the study of nanomechanical resonators, ultra-sensitive measurement techniques are crucial. However, if the measurement sensitivity approaches quantum-mechanical limits, the back-action of the detector on the resonator cannot be neglected. If the back-action is strong enough, the corresponding instability can create self-sustained oscillators in the resonator. Here we demonstrate that a torsional mechanical resonator, which contains a direct current SQUID displacement detector, leads to this effect. We find that the Lorentz-force back-action can be so large that, in combination with complex nonlinear Josephson dynamics, it generates intrinsic self-sustained oscillations. The flux quantization limit of the maximum oscillation amplitude is exploited to calibrate the displacement resolution, which is shown to be below the standard quantum limit. The suspended torsional SQUID provides an interesting platform to study on-chip laser-like physics in an electromechanical system that can be controlled by both a flux and current bias. Self-sustained oscillations (SSOs) are distinct from the forced motion of a resonator because the oscillation period does not depend on the frequency of the driving force. Resonators in the SSO regime typically produce signals with a spectral line width, which is narrower than the intrinsic line width of the resonator. The reduced line width enhances the sensitivity of resonance-based force-gradient sensors [1] . On the other hand, these oscillations are not desirable in experiments that require observation of very small displacements, such as those induced by gravitational waves [2] and quantum-mechanical zero-point fluctuations [3] , [4] , [5] . Therefore, understanding the origin and behaviour of the SSO is essential. Self-sustained mechanical oscillations are induced by strong feedback between mechanical motion and the detector [6] , [7] , [8] . This can be engineered externally, if the amplifier is added as an external element in the circuit [9] , [10] . An example of such an oscillator is an electronic amplifier, which applies a magnetomotive feedback force to a mechanical resonator [9] . In contrast, the feedback can also be due to intrinsic detector–resonator interaction [11] , [12] . For example, an optomechanical oscillator can be sustained by radiation pressure back-action [11] . In electromechanical systems, mesoscopic electronics are an important class of detectors. Devices such as the Atomic Point Contact [13] and the Single Electron Transistor [14] , [15] greatly enhance both the displacement resolution and the back-action. Despite considerable theoretical interest [16] , [17] , direct observation of sufficiently strong back-action and intrinsic SSO has not been reported in a mesoscopic electromechanical system. The displacement detector in this letter consists of a mechanical resonator, which contains a direct current (dc) Superconducting QUantum Interference Device (SQUID) loop. By virtue of its high flux-to-voltage responsivity, the SQUID enables accurate measurement of the vibrations of the resonator. In contrast to previous work where only part of the loop was suspended [18] , here we suspend the entire SQUID, forming a torsional resonator. We have previously studied the dynamic back-action that the SQUID exerts on an embedded resonator when the resonator displacement causes only small flux variations [19] . Here we show that the torsional resonator is more strongly coupled to the SQUID. Specifically, we find that the behaviour on the upward and the downward flank of the voltage-flux curve is strikingly different. Although the upward flank shows the usual driven motion, the data for the downward flank display SSOs, as substantiated by the large amplitude, sharp profile, and, most importantly, the ring-shaped distribution of the waveform amplitude around zero. The mechanical vibrations cause large flux oscillations, on the order of a flux quantum, Ф 0 = h /2 e =2 fWb. Voltage noise spectra The torsional dc SQUID ( Fig. 1a ) is fabricated from an InAs-AlGaSb heterostructure, which is epitaxially grown on a GaAs [111a] substrate (see Methods ). Measurements are performed at 20 mK in vacuum. To detect the out-of-plane motion of the suspended SQUID loop, a parallel magnetic field is applied ( Fig. 1a ). The field transduces the change in loop area into a change in magnetic flux. The SQUID transport characteristics are shown in Fig. 1c (voltage-current) and its inset (voltage-flux). For the measurements below, the SQUID is operated in a feedback loop that is set to the blue dots in Fig. 1c . Note that the SQUID can be biased to either the upward or the downward flank of the voltage-flux curve (see Methods ). 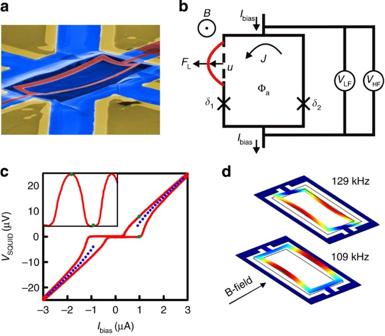Figure 1: Device characteristics. (a) Colourized scanning electron microscope image of the suspended 95 × 40 μm2SQUID (red) at an angle of 80 degrees to the substrate (blue). The Josephson junctions are located in the loop. (b) Schematic overview of the SQUID geometry and parameters. The resonator is represented by the deformed section of the loop marked in red. In reality, the displacement is out-of-plane and the magnetic field in-plane; in the schematics, motion for convenience is represented as in-plane.B,Ib, and Фaare the applied magnetic field, bias current and magnetic flux, respectively. The two junctions have phaseδ1,2of the superconducting order parameter,uis the deflection of the resonator coordinate from its equilibrium position,Jis the circulating current around the loop andFLis the Lorentz force on the resonator. The voltage across the loop is measured using a low-frequency (LF, <1 kHz) and a high-frequency amplifier (HF, >1 kHz). The arrows point in the positive direction of the respective variables. (c) Measured SQUID voltage versus bias current. For each bias current in the main plot, a voltage-flux trace is measured over at least one flux quantum (inset). The red lines in the main figure show the minimum and maximum voltages (green dots) obtained from each trace. The blue dots mark the bias at which the resonator measurements ofFig. 2are taken. (d) Finite-element simulation of the two lowest mechanical resonance modes for a geometrically symmetrical SQUID. Red denotes high displacement amplitude, whereas blue denotes a small displacement. Figure 1: Device characteristics. ( a ) Colourized scanning electron microscope image of the suspended 95 × 40 μm 2 SQUID (red) at an angle of 80 degrees to the substrate (blue). The Josephson junctions are located in the loop. ( b ) Schematic overview of the SQUID geometry and parameters. The resonator is represented by the deformed section of the loop marked in red. In reality, the displacement is out-of-plane and the magnetic field in-plane; in the schematics, motion for convenience is represented as in-plane. B , I b , and Ф a are the applied magnetic field, bias current and magnetic flux, respectively. The two junctions have phase δ 1,2 of the superconducting order parameter, u is the deflection of the resonator coordinate from its equilibrium position, J is the circulating current around the loop and F L is the Lorentz force on the resonator. The voltage across the loop is measured using a low-frequency (LF, <1 kHz) and a high-frequency amplifier (HF, >1 kHz). The arrows point in the positive direction of the respective variables. ( c ) Measured SQUID voltage versus bias current. For each bias current in the main plot, a voltage-flux trace is measured over at least one flux quantum (inset). The red lines in the main figure show the minimum and maximum voltages (green dots) obtained from each trace. The blue dots mark the bias at which the resonator measurements of Fig. 2 are taken. ( d ) Finite-element simulation of the two lowest mechanical resonance modes for a geometrically symmetrical SQUID. Red denotes high displacement amplitude, whereas blue denotes a small displacement. Full size image The resonator displacement is detected by measuring the SQUID output voltage. The eigenmodes of the torsional SQUID are found by driving a piezo actuator with a sinusoidal voltage and measuring the SQUID voltage at the same frequency. The lowest mechanical resonance modes are found at 109 and 129 kHz. The quality factor is extracted from a fit to the frequency response, yielding a quality factor of around 7,000 for both modes. Finite-element simulations show the nature of the eigenmodes to be a combination of flexural and torsional motion ( Fig. 1d ). The lowest mode exhibits in-phase motion of the two arms, but is still detectable due to some arm asymmetry. The piezo drive is used only to locate the eigenmodes and is turned off for the measurements below. Voltage noise spectra of the two lowest modes are shown in Fig. 2a . The spectra are measured on the upward flank (blue data) and the downward flank (red data) of the voltage-flux curve. Compared with the spectra on the upward flank, the spectra on the downward flank are much sharper, and the total power (the area under the resonance peaks) increases strongly, indicating oscillations with high amplitude. 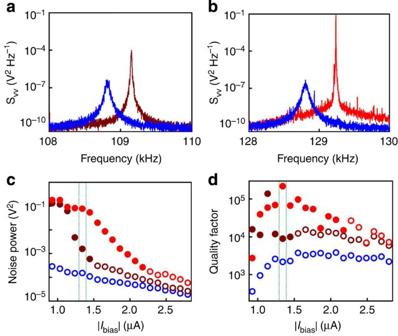Figure 2: Spectral measurements. (a) Power spectral density of the 109 kHz mode atIbias=+1.4 μA. The blue spectrum is due to thermal motion of the mode, measured on the positive (upward) flankVФ>0. On the negative (downward) flankVФ<0, the noise peak (in red) sharpens and increases in amplitude by four orders of magnitude, indicative of SSOs. The frequency shift between the two spectra is due to the SQUID back-action. (b) The spectra of the 129 kHz mode are measured atIbias=−1.4 μA. The behaviour is similar to the 109 kHz mode, with SSO occurring on the same flankVФ<0. (c) Integrated noise power of the resonance peaks as a function of bias current. Red points are measured for negative bias currents with solid circles identifying the SSO regime; dark red: 109 kHz; light red: 129 kHz. Open circles represent the non-SSO regime. The data points for the spectra of figures a and b are marked by the green window. On the positive flankVФ>0, no SSO is observed and the noise power is due to thermal motion (open blue circles). Only the 109-kHz thermal data is shown, as the 129-kHz data, measured on the oppositeV–Ф flank, is nearly identical. (d) Effective quality factor obtained from fits to the noise spectra. The thermal spectra on the positive flankVФ>0 have the lowestQvalues, whereas the 129-kHz mode reaches values >105in the SSO regime. Figure 2c shows the power and the effective quality factor as a function of the bias current, respectively. The effective quality factor Q is defined as the full-width at half-maximum of the peaks divided by the peak frequency [9] . The high amplitudes for the 109-kHz mode occur at positive bias, near the maximum critical current ( Fig. 1c ), whereas the high amplitudes for the 129-kHz mode occur at negative bias current. Thus, the modes do not oscillate with high amplitude simultaneously, and apparently the large motion of one mode disrupts the motion of the other. Similar competition was also observed between cantilever modes in optomechanical cavities [6] and between cavity modes in lasers [20] . Figure 2: Spectral measurements. ( a ) Power spectral density of the 109 kHz mode at I bias =+1.4 μA. The blue spectrum is due to thermal motion of the mode, measured on the positive (upward) flank V Ф >0. On the negative (downward) flank V Ф <0, the noise peak (in red) sharpens and increases in amplitude by four orders of magnitude, indicative of SSOs. The frequency shift between the two spectra is due to the SQUID back-action. ( b ) The spectra of the 129 kHz mode are measured at I bias =−1.4 μA. The behaviour is similar to the 109 kHz mode, with SSO occurring on the same flank V Ф <0. ( c ) Integrated noise power of the resonance peaks as a function of bias current. Red points are measured for negative bias currents with solid circles identifying the SSO regime; dark red: 109 kHz; light red: 129 kHz. Open circles represent the non-SSO regime. The data points for the spectra of figures a and b are marked by the green window. On the positive flank V Ф >0, no SSO is observed and the noise power is due to thermal motion (open blue circles). Only the 109-kHz thermal data is shown, as the 129-kHz data, measured on the opposite V –Ф flank, is nearly identical. ( d ) Effective quality factor obtained from fits to the noise spectra. The thermal spectra on the positive flank V Ф >0 have the lowest Q values, whereas the 129-kHz mode reaches values >10 5 in the SSO regime. 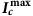Figure 3: Time-resolved measurements of the SQUID voltage atIb=−. (a) Measured oscillator waveform during startup and ring-down (red). The startup follows the step response of a negative-feedback amplifier (left blue line), and the ring-down follows the exponential decay, which is expected for a harmonic oscillator withQ=7,000 (right blue line). The voltage is measured using a high-mobility-electron transistor (HEMT). (b) Oscillation frequency during the same startup and ring-down. When theVФflank is switched, the frequency shifts to its new value within a few milliseconds. In contrast, the amplitude of the oscillator as seen inareacts more slowly. (c) Measured waveforms of the 129-kHz SSO atIb=−(red) and of the thermal motion on the otherVФflank (blue). The oscillator waveform contains higher harmonics due to the non-linear response of the SQUID detector. (d) Simulated oscillator waveform, with the peak-voltage and peak-flux oscillation amplitude as free parameters. The flux oscillation amplitude is found to be 0.3 Ф0and the peak–peak voltage amplitude is 0.75 V. Full size image Time record Figure 3a shows the measured and processed time record of the SQUID voltage due to the 129-kHz mode after switching the SQUID from the upward flank to the downward flank (see Methods ). The ring-up timescale is longer than the ring-down because the ring-up occurs with a high quality factor ( Fig. 2d ), whereas the ring-down is faster because of the lower quality factor. The individual oscillations in the saturated range of Fig. 3a are shown in Fig. 3c . For comparison, the much smaller waveform at the upward flank is also shown. Note that on this timescale, both waveforms have a constant amplitude and phase. This is expected even for random thermal motion because the intrinsic quality factor of the 129-kHz mode (7,000) is such that the amplitude and phase are randomized on a timescale much larger than the one used in Fig. 3c . Figure 3: Time-resolved measurements of the SQUID voltage at I b =− . ( a ) Measured oscillator waveform during startup and ring-down (red). The startup follows the step response of a negative-feedback amplifier (left blue line), and the ring-down follows the exponential decay, which is expected for a harmonic oscillator with Q =7,000 (right blue line). The voltage is measured using a high-mobility-electron transistor (HEMT). ( b ) Oscillation frequency during the same startup and ring-down. When the V Ф flank is switched, the frequency shifts to its new value within a few milliseconds. In contrast, the amplitude of the oscillator as seen in a reacts more slowly. ( c ) Measured waveforms of the 129-kHz SSO at I b =− (red) and of the thermal motion on the other V Ф flank (blue). The oscillator waveform contains higher harmonics due to the non-linear response of the SQUID detector. ( d ) Simulated oscillator waveform, with the peak-voltage and peak-flux oscillation amplitude as free parameters. The flux oscillation amplitude is found to be 0.3 Ф 0 and the peak–peak voltage amplitude is 0.75 V. Full size image Waveforms To study the amplitude and phase drift, the waveform behaviour on a longer timescale is measured and shown in a phase plot. In such a plot, the in-phase and quadrature components of the waveform are extracted (see Methods ), so that the amplitude and phase of the waveform can be observed over many oscillation periods. 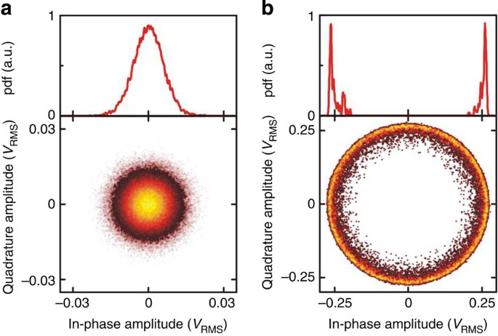Figure 4: Phase plots of the 129 kHz waveforms measured over a period of 2,000 s. Colours indicate the probability of observing a given amplitude and phase (probability density function (pdf)), where yellow and red indicate high and low probability, respectively. White indicates zero incidence. (a) Phase plot of the low-amplitude waveform (top graph is a horizontal line trace through zero). Both the amplitude and the phase have a Gaussian distribution around zero, a signature of random, thermal motion. (b) Phase plot of the high-amplitude waveform. The amplitude of the oscillation is well defined, and phase noise dominates a signature of steady-state oscillation. Note that the horizontal scale ofbis almost an order of magnitude larger than that ofa, consistent with the high- and low-amplitude waveforms measured in real time. Figure 4a shows the phase plot of the low-amplitude waveform of Fig. 3c over 2,000 s. A noiseless oscillator has a phase plot, which consists of a single point, or in other words, it is a stable phasor. Amplitude noise causes broadening in the direction of the phasor, whereas phase noise causes broadening in the tangential direction. If the resonator displacements are due to thermal force noise, the phase plot consists of a Gaussian distribution, which is symmetrical and centred around zero amplitude. The phase plot in Fig. 4a has such a distribution, confirming that the blue waveform of Fig. 3c is due to thermal motion. We have verified that the other blue spectra in Fig. 2 have the same characteristic Gaussian distribution, and we therefore refer to these as thermal spectra. Figure 4: Phase plots of the 129 kHz waveforms measured over a period of 2,000 s. Colours indicate the probability of observing a given amplitude and phase (probability density function (pdf)), where yellow and red indicate high and low probability, respectively. White indicates zero incidence. ( a ) Phase plot of the low-amplitude waveform (top graph is a horizontal line trace through zero). Both the amplitude and the phase have a Gaussian distribution around zero, a signature of random, thermal motion. ( b ) Phase plot of the high-amplitude waveform. The amplitude of the oscillation is well defined, and phase noise dominates a signature of steady-state oscillation. Note that the horizontal scale of b is almost an order of magnitude larger than that of a , consistent with the high- and low-amplitude waveforms measured in real time. Full size image In contrast, Fig. 4b shows that the high-amplitude waveform of Fig. 3c has a ring-shaped distribution around zero. The amplitude shows an asymmetric peak around a non-zero mean, and the noise in the amplitude direction is much smaller than the mean value. The phase, on the other hand, goes through all angles. This behaviour is expected for resonators that experience nonlinear negative feedback [21] : the oscillation amplitude grows until the SQUID can no longer increase its back-action on the resonator, causing the amplitude to settle on a steady-state value. The phase of the oscillator has no restrictions and is therefore allowed to drift freely, leading to a ring-shaped phase plot. Such a plot is thus a clear signature of SSO. The SQUID-resonator back-action is provided by the Lorentz force, which acts on the resonator and modifies the effective spring constant and effective damping. This Lorentz force is created by the external magnetic field and is proportional to the current circulating through the SQUID loop [19] . In turn, the current depends non-linearly on the magnetic flux through the loop, which is sensitive to the displacement of the resonator. The back-action can be probed by investigating the shifts of the frequency and the quality factor of the resonator at different biasing conditions (magnetic flux and bias current). For the device used in the experiments, the coupling between the SQUID and the resonator is sufficiently strong to cause negative damping of the mechanical resonator close to the critical current. This implies that the resonator gains energy each oscillation cycle instead of losing it, which causes it to exhibit SSO. Quantitative estimates for the back-action are presented in Methods section, and a simplified model is given in Supplementary Methods . Responsivity To calibrate the displacement responsivity of the SQUID, we use the waveform of the SSO ( Fig. 3c ) and the fact that the SQUID voltage response is Ф 0 periodic. This periodicity serves as the calibration standard: From the applied magnetic field and the dimensions of the resonator, we calculate that a resonator displacement of 0.27 nm relates to a flux change of one quantum. The waveform is fit to the flux response shown in Fig. 1c , and we find a flux oscillation amplitude of 0.3 Ф 0 . The fitted waveform is shown in Fig. 3d . From the fit, we get a responsivity of 6.1 μV fm −1 . This calibration method provides a fast, accurate alternative to the standard thermal calibration [18] , [22] , which does not work here because of the large back-action. The responsivity, combined with the output voltage noise floor of the amplifier (4.1 μV ), spring constant (1.5 N m −1 ) and effective bandwidth (29 Hz) of the mechanical resonator, yields a detector resolution of 3.6 fm, which is below the standard quantum limit of 5.3 fm. Detailed calculations are provided in Supplementary Methods . The intrinsic nature of the SSO, combined with the large operating bandwidth of the Josephson junctions, means that embedded nano-scale resonators with GHz frequencies (for example, carbon nanotubes) may also exhibit SSO without any external feedback. Future research must be directed at understanding how the possibility of SSO affects applications of SQUID-based electronics for ultra-sensitive position detection [4] , [5] , for quantum state transduction [3] , for studies of frequency entrainment [23] , [24] , [25] and sensitive force-gradient detection [1] . The observation of SSO suggests that a torsional SQUID oscillator may also be a good candidate to observe laser-like physics with phonons previously predicted theoretically for other nanomechanical systems [16] , [17] , [26] . Both the applied flux and current bias can be used as control parameters, providing access to a wide parameter range. Sample preparation The dc SQUID ( Fig. 1a ) is fabricated from an InAs-AlGaSb heterostructure, which is epitaxially grown on a GaAs [111a] substrate. The SQUID ring (95 × 40 μm 2 ) is formed by evaporation of 100 nm of Nb on the InAs surface. A 250-nm long gap in each of the 4.5-μm wide arms forces current to flow through the 42.5-nm thick InAs layer, thereby forming superconductor-normal metal-superconductor-type Josephson junctions. Titanium-gold contacts are evaporated on the leads for connection to off-chip electronics. Around the SQUID, the InAs and AlGaSb layers are removed by a BCl 3 -reactive ion etch to define the resonator and provide electronic insulation. The GaAs underneath the resonator is removed by an isotropic ammonia wet etch so that the SQUID is almost completely suspended; only the current leads anchor the SQUID to the substrate. This geometry allows the SQUID loop to perform flexural and torsional motion. The substrate with the SQUID is glued on top of a piezoelectric transducer, which is used to excite the eigenmodes of the resonator. This ensemble is mounted inside a dilution refrigerator and is operated at its base temperature of 20 mK in high vacuum. Experimental details Stable operation is achieved by operating the SQUID in a low-frequency feedback loop (<1 kHz), which adjusts the applied flux to maintain a constant setpoint voltage V SP . Note, that for a given bias current and voltage setpoint, the feedback loop can be set to lock either to the upward or the downward flank of the V– Ф curve (inset of Fig. 1c ). These are denoted by V Ф ≡ ∂ V / ∂ Ф>0 and V Ф <0, respectively. The magnetic field is applied to the SQUID by a superconducting solenoid magnet, whereas the magnetic flux through the loop is fine-tuned with a small coil near the device. The voltage generated by the resonator motion is measured using a high-electron-mobility transistor amplifier at the 1 K stage of the dilution refrigerator. SQUID transport characterization To determine the working point of the SQUID, its electronic transport characteristics are first measured. Figure 1c shows voltage-current and voltage-flux traces for the SQUID at an applied magnetic field of B =+80 mT, which is used throughout this work. The SQUID output voltage is zero at low-bias currents and behaves Ohmically at bias currents well above the critical current. The maximum critical current is =1.1 μA (0.55 μA per junction), and the normal-state resistance of the two junctions in parallel is R =8Ω. The voltage is most sensitive to the magnetic flux in the transition region between superconducting and Ohmic behaviour. The inset of Fig. 1c shows the output voltage of the SQUID when the magnetic field is swept. The voltage is periodic with a period of one flux quantum. The linear response of the SQUID is largest near the middle of the upward and the downward flank of the V– Ф curve, and this is where we bias the SQUID (blue points in Fig. 1c ). Torsional SQUID displacement The displacement u of a given resonance mode is defined as the root-mean-squared displacement of that mode, integrated over the resonator length. The amplitude u of each normal mode is thus determined through the spatial profile of the mode (see Poot and van der Zant [27] for more details). This definition ensures that the spring constant equals k R = m R , where m R is the total mass of the resonator and ω R is the resonance frequency. The change in magnetic flux for a given displacement is then found by calculating the change in area of the inner loop in the plane perpendicular to the magnetic field direction. This results in a flux change ∂ Ф/ ∂ u = aB per unit deflection. Here, is the length of the resonator, perpendicular to the magnetic field direction, and a is a geometrical factor that depends on the shape of the resonance mode and the orientation of the magnetic field. For the two lowest modes, we estimate a ≈1. For two dissimilar arms, the geometrical factor is effectively that of a single-beam resonator, for which the geometrical factor is 0.91 ( [18] ). Distortions of the loop may also have a minor influence on the value of a , therefore we have taken a ≈1 in the remainder of the manuscript. Waveform data processing For the data in Fig. 3 , the mean of the measured waveform has been subtracted. In addition, the waveform has been filtered such that it only contains the signal in a bandwidth of 1 kHz around the 129-kHz resonance peak and its harmonics. Note that the full-width half-maximum of the mechanical signal is <20 Hz. The phase plots in Fig. 4 are processed from waveforms such as those in Fig. 3c , recorded over a longer timescale (2,000 s). To extract the amplitude and the phase of the measured waveform, the time record is multiplied by pure cosine and sine waveforms at the oscillation frequency. The resulting time series are passed through a moving-average filter to eliminate spurious frequency components. This yields the in-phase and quadrature (90 degrees out-of-phase) amplitudes of the waveform, from which the phase plots of Fig. 4 are constructed. SQUID-induced frequency shift In addition to the resonator damping shifts, the SQUID back-action also shifts the resonance frequency. Supplementary Fig. S1 shows the frequency shift as a function of applied bias current. The instantaneous frequency is extracted from the waveform by filtering out the harmonics of the 129-kHz signal and locating the times at which the resulting waveform crosses the zero volt axis. The frequency is then calculated by taking the reciprocal of the time between two adjacent zero-crossings. The trend is similar to what was observed for the SQUIDs with the embedded MHz beam resonators in previous work [19] . In that work, the back-action strength was quantified by the dimensionless coupling parameter Δ f for the frequency shift and Δ Q for the quality factor: where ω 0 and Q 0 are the intrinsic resonance frequency and quality factor of the mechanical resonator, and R is the resistance of Josephson junctions. The frequency shift relative to the intrinsic resonance frequency is stronger for the torsion resonator than for the beam resonator. This is consistent with the increased coupling parameter; Δ f =1 × 10 −2 for the torsion resonator versus Δ f =4 × 10 −4 for the beam resonator of ref. 19 . It is interesting to examine the time it takes for the resonance frequency to shift after the SQUID switches flanks and compare it to the ring-up and down times. The resonance frequency shifts with SQUID bias due to dynamical back-action [19] . Figure 3b shows the frequency as a function of time. There, the frequency shifts by 1 kHz within a few milliseconds of switching the flanks. The step response of the frequency is thus much faster than the amplitude step response. This also implies that the time it takes to switch the SQUID between the positive and negative flanks is less than a few milliseconds. Back-action estimates To quantify the back-action in the torsional SQUID, we use the analysis presented in ref. 19 . In that paper, the dynamical back-action on the resonator is modelled as a change in the effective damping and resonance frequency of the mechanical resonator due the current that circulates around the SQUID loop. The total damping of the resonator was written as where γ 0 is the intrinsic resonator damping. The dimensionless gain factor j φ˙ is tunable by the applied bias. Other than this, j φ˙ only depends on the inductance and capacitance of the SQUID, which are the same as for the device in Poot [19] . Its maximum value was calculated to be 500. The dimensionless coupling parameter Δ Q is independent of the bias of the SQUID but depends on the parameters of both the SQUID and the resonator. Negative damping occurs when the product j φ˙ Δ Q is greater than one. For the sample with the embedded beam resonator [19] , the coupling parameter Δ Q =2.8 × 10 −4 , which means that the maximum product max( j φ˙ Δ Q )=0.14 was too small to achieve negative damping. The increased length of the torsion SQUID resonator (95 versus 50 μm) and its decreased spring constant (1.5 versus 100 N m −1 ) result in Δ Q =2.2 × 10 −3 . This coupling is almost an order of magnitude larger than that of the beam-SQUID and is sufficiently strong to induce negative damping, in agreement with our observations. How to cite this article: Etaki, S. et al . Self-sustained oscillations of a torsional SQUID resonator induced by Lorentz-force back-action. Nat. Commun. 4:1803 doi:10.1038/ncomms2827 (2013).